Inflammation-driven carcinogenesis is mediated through STING Chronic stimulation of innate immune pathways by microbial agents or damaged tissue is known to promote inflammation-driven tumorigenesis by mechanisms that are not well understood. Here we demonstrate that mutagenic 7,12-dimethylbenz(a)anthracene (DMBA), cisplatin and etoposide induce nuclear DNA leakage into the cytosol that intrinsically activates stimulator of interferon genes (STING)-dependent cytokine production. Inflammatory cytokine levels are subsequently augmented in a STING-dependent extrinsic manner by infiltrating phagocytes purging dying cells. Consequently, STING −/− mice, or wild-type mice adoptively transferred with STING −/− bone marrow, are almost completely resistant to DMBA-induced skin carcinogenesis compared with their wild-type counterparts. Our data establish a role for STING in the control of cancer, shed significant insight into the causes of inflammation-driven carcinogenesis and may provide a basis for therapeutic strategies to help prevent malignant disease. The innate immune response is essential for protection of the host against microbial infection, although chronic stimulation of these pathways can cause unwarranted inflammatory disease including systemic lupus erythematosus (SLE) and even cancer [1] , [2] , [3] . While the toll-like receptor and RIG-I-like (RLR) pathways have been clearly shown to be important in facilitating innate immune signalling processes in response to pathogens, they have not been found to be notably responsible for manifesting inflammatory disorders induced by self-DNA [4] . Recently, however, a cellular sensor referred to as STING (for stimulator of interferon (IFN) genes) has been shown to control innate immune gene activation in response to cytosolic DNA generated by DNA pathogens, necrotic or inappropriately apoptosed cells [5] , [6] , [7] . Whereas STING is essential for production of type I IFN following pathogen infection of the cell, chronic STING activity has been found to lead to lethal inflammatory disease in model systems and may be responsible for Aicardi–Goutieres syndrome (AGS) and plausibly other disorders in human patients [5] , [8] . DMBA induces cytokine production in a STING-dependent manner Inflammation triggered by infectious disease or environmental carcinogens is also considered to play a key role in tumour development, although the mechanisms remain to be fully elucidated [1] , [2] . Given this and the importance of STING in mediating cytokine production, we therefore queried the plausible role of STING in inflammation-driven carcinogenesis. To facilitate this, we utilized the carcinogen 7,12-dimethylbenz(a)anthracene (DMBA), a polyaromatic hydrocarbon (PAH) known to induce cutaneous tumours when applied to the skin of mice [9] . PAHs are currently classified as human mutagens and have been shown to have a carcinogenesis effect in humans [10] . DMBA is known to activate cytokine-driven MyD88 signalling and tumour necrosis factor alpha (TNFα) production, which facilitates tumorigenesis, although the initiating responsible pathway remains unknown [11] , [12] . We thus treated wild-type (WT) mouse embryonic fibroblasts (MEFs) or STING-deficient MEFs (SKO) with DMBA and examined cytokine production by these cells. Principally, we observed that DMBA clearly triggered STING translocation from the endoplasmic reticulum (ER) to perinuclear, non-ER microsome compartments in the cells ( Fig. 1a ). The translocation of STING via autophagy is essential to invoke STING-dependent signalling [13] , [14] . We further demonstrated that DMBA induced STING phosphorylation, indicated by an increase in the molecular weight of STING [14] , an event also required for STING activity ( Fig. 1a ). Further, microarray analysis of DMBA-treated WT cells indicated a wide variety of cytokine and chemokine production, including IL1 , ICAM1 , IL11 , PTGES and TNFα , which are known proinflammatory agents ( Fig. 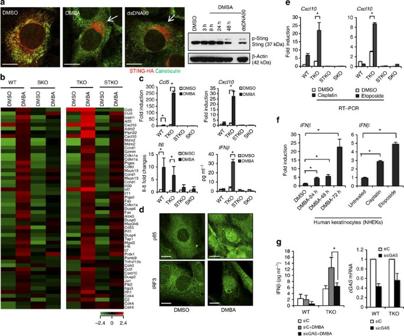Figure 1: The role of STING in DMBA-induced cytokine production. (a) WT MEFs expressing STING-HA were either transfected with 3 μg ml−1of dsDNA90 for 3 h or treated with 20 μg ml−1of DMBA. DMSO treatment was included as control. Using HA antibody for STING and anti-calreticulin for ER marker, immunofluorescence microscopy analysis was performed 48 h after DMBA treatment (left, original magnification at × 1,260; bar size, 10 μm) and immunoblot analysis was performed at the designated time points (right), (also seeSupplementary Fig. 10). p-Sting, phosphorylated STING. (b) Gene array analysis of WT, TKO, STKO and SKO MEFs treated with DMBA at 20 μg ml−1or DMSO as control for 48 h. Highest variable inflammation-related genes are shown. Rows represent individual genes; columns represent individual samples. Pseudo-colours indicate transcript levels below (green), equal to (black) or above (red) the mean. Scale represents the intensity of gene expression (log2 scale ranges between −2.4 and 2.4). (c) Quantitative PCR (qPCR) analysis and IFNβ ELISA assay of MEFs treated with DMBA same as inb. (d) Immunofluorescence microscopy analysis of p65 and IRF3 in WT MEFs treated with DMBA same as inb. Original magnification, × 1,260; bar size, 10 μm. (e) qPCR analysis of WT, TKO, STKO and SKO MEFs treated with 10 μM of cisplatin or 250 μM of etoposide for 48 h. DMSO treatment was included as controls. (f) qPCR analysis ofIFNβmessenger RNA in human keratinocytes treated with 20 μg ml−1of DMBA for 24, 48 or 72 h or with 10 μM of cisplatin or 250 μM of etoposide for 48 h. (g) WT and TKO MEFs were transfected with cGAS or control small interfering RNA (siRNA) for 48 h followed by DMBA treatment same as inb, and were then subjected to the IFNβ ELISA assay.cGASexpression level after siRNA treatment was determined by qPCR. Data are representative of at least two independent experiments. Error bars indicate s.d. *P<0.05, Student’st-test. WT;Sting+/+Trex1+/+, SKO;Sting−/−Trex1+/+, TKO;Sting+/+,Trex1−/−, STKO;Sting−/−,Trex1−/−. 1b ; Supplementary Table 1 ). Significantly, the induction of these genes by DMBA was markedly reduced in SKO MEFs, indicating that their production involved the STING pathway ( Fig. 1b ; Supplementary Table 1 ). To investigate further, we similarly treated MEFs lacking functional DNaseIII (Trex1) expression with DMBA. Trex1 may function, at least in part, to degrade STING agonists such as leaked DNA in the cytoplasm, since loss of Trex1 function in mice causes STING-dependent lethal inflammatory diseases [8] , [15] , [16] . Mutations in Trex1 have also been found in patients with AGS and severe SLE [17] . We postulated that the effects of DMBA may be profoundly accentuated in the absence of Trex1. This analysis indeed confirmed that DMBA-treated MEFs lacking Trex1 (TKO) had even more augmented cytokine production compared with WT MEFs ( Fig. 1b ; Supplementary Table 1 ). This was verified using quantitative real-time PCR (qPCR) analysis and enzyme-linked immunosorbent assay (ELISA) to demonstrate a comprehensive increase in type I IFN production in DMBA-treated cells lacking Trex1, events that were almost completely suppressed in the absence of STING ( Fig. 1c ; Supplementary Fig. 1a,b ). Accordingly, we observed STING-dependent activation and nuclear translocation of both NF-κB and IRF3 in DMBA-treated WT and TKO MEFs, but not in cells lacking STING ( Fig. 1d ; Supplementary Fig. 1c–f ). 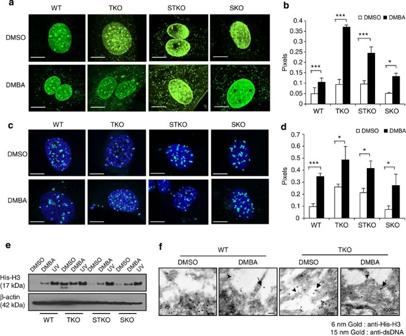Figure 2: Cytoplasmic nucleosome production in DMBA-treated cells is independent of STING. (a) Fluorescence microscopy analysis of anti-dsDNA staining (a,b) and fluorescentin situhybridization (FISH) with mouse centromere probe (c,d) in WT, TKO, STKO and SKO MEFs treated with DMBA at 20 μg ml−1or DMSO as control for 48 h. Representative images are shown at × 1,260; bar size, 10 μm (a,c), and ratio of cytoplasm to nucleus anti-dsDNA pixels fromaand FISH pixels fromcwas quantitated using Leica LAS AF software (b,d). (e) Immunoblot analysis of histone H3 in cytoplasmic extraction from MEFs treated with DMBA same as inaor ultraviolet at 120 mJ cm−2followed by 24-h incubation (also seeSupplementary Fig. 10). (f) Electron microscopy analysis of histone H3 and dsDNA gold staining in WT and TKO MEFs treated with DMBA same as ina. Arrows indicate gold particles in cytoplasm. Images were shown at original magnification, × 100,000; bar size, 100 nm. Data are representative of at least two independent experiments. Error bars indicate s.d. *P<0.05, ***P<0.001, Student’st-test. Given this, we next considered whether other DNA adduct-forming agents, including cisplatin and etoposide, were similarly capable of stimulating STING-dependent cytokine activation comparable to DMBA ( Supplementary Table 2 ) [18] . This analysis, carried out on MEFs and primary human keratinocytes, confirmed that a variety of DNA-damaging agents are able to stimulate cytokine production in a STING-dependent manner ( Fig. 1e,f ; Supplementary Fig. 2a–f ). Similar to loss of STING, we observed that knockdown of cGAS, a cyclic guanosine monophosphate–adenosine monophosphate synthase that produces non-canonical cyclic dinucleotides capable of activating STING [19] , also greatly reduced the production of inflammatory cytokines triggered by DMBA as well as by other DNA-damaging agents, such as cisplatin and camptothecin ( Fig. 1g ; Supplementary Fig. 2g,h ). Thus, the mutagens, DMBA, cisplatin and etoposide, generate intrinsic inflammatory effects through the activation of STING-dependent signalling. Figure 1: The role of STING in DMBA-induced cytokine production. ( a ) WT MEFs expressing STING-HA were either transfected with 3 μg ml − 1 of dsDNA90 for 3 h or treated with 20 μg ml − 1 of DMBA. DMSO treatment was included as control. Using HA antibody for STING and anti-calreticulin for ER marker, immunofluorescence microscopy analysis was performed 48 h after DMBA treatment (left, original magnification at × 1,260; bar size, 10 μm) and immunoblot analysis was performed at the designated time points (right), (also see Supplementary Fig. 10 ). p-Sting, phosphorylated STING. ( b ) Gene array analysis of WT, TKO, STKO and SKO MEFs treated with DMBA at 20 μg ml − 1 or DMSO as control for 48 h. Highest variable inflammation-related genes are shown. Rows represent individual genes; columns represent individual samples. Pseudo-colours indicate transcript levels below (green), equal to (black) or above (red) the mean. Scale represents the intensity of gene expression (log2 scale ranges between −2.4 and 2.4). ( c ) Quantitative PCR (qPCR) analysis and IFNβ ELISA assay of MEFs treated with DMBA same as in b . ( d ) Immunofluorescence microscopy analysis of p65 and IRF3 in WT MEFs treated with DMBA same as in b . Original magnification, × 1,260; bar size, 10 μm. ( e ) qPCR analysis of WT, TKO, STKO and SKO MEFs treated with 10 μM of cisplatin or 250 μM of etoposide for 48 h. DMSO treatment was included as controls. ( f ) qPCR analysis of IFNβ messenger RNA in human keratinocytes treated with 20 μg ml − 1 of DMBA for 24, 48 or 72 h or with 10 μM of cisplatin or 250 μM of etoposide for 48 h. ( g ) WT and TKO MEFs were transfected with cGAS or control small interfering RNA (siRNA) for 48 h followed by DMBA treatment same as in b , and were then subjected to the IFNβ ELISA assay. cGAS expression level after siRNA treatment was determined by qPCR. Data are representative of at least two independent experiments. Error bars indicate s.d. * P <0.05, Student’s t -test. WT; Sting +/+ Trex1 +/+ , SKO; Sting −/− Trex1 +/+ , TKO; Sting +/+ , Trex1 −/− , STKO; Sting −/− , Trex1 −/− . Full size image DMBA causes cytoplasmic DNA leakage independent of STING STING is known to control the induction of cytokines by aberrant cytosolic DNA species [6] , [7] . We noted that it has previously been shown that cell death invoked by etoposide can cause nucleosome leakage into the cytoplasm, plausibly generated by single- or double-strand breaks of DNA promoted by DNA adduct formation [20] . The presence of nuclear DNA in the cytoplasm could conceivably activate the STING pathway and generate cytokine production. Initially, we observed that DMBA-treated MEF cells underwent slightly more cell death over a period of 3 days, as determined by trypan blue analysis and Annexin V staining ( Supplementary Fig. 3a,b ). We concomitantly examined DMBA-treated MEFs and examined the cells for the presence of cytoplasmic DNA. This approach showed significant DNA leakage in the cytoplasm of DMBA-, cisplatin- or etoposide-treated MEFs, but not mock-treated MEFs, as determined by fluorescence in situ hybridization analysis, anti-double-stranded DNA (dsDNA) antibody as well as PicoGreen staining (a dsDNA stain), ( Fig. 2a–d ; Supplementary Fig. 3c,d ). A similar effect was seen in MEF cells lacking STING, indicating that this event was STING independent ( Fig. 2a–d ; Supplementary Fig. 3c,d ). To extend this analysis further, we examined, by two approaches, whether DMBA-treated cells also exhibited an increase in the presence of extranuclear histones. As determined by fractionation analysis of cytoplasmic cell extracts treated with or without DMBA or ultraviolet irradiation, DMBA-treated MEFs indeed displayed the presence of cytoplasmic histones (histone H3) ( Fig. 2e ). Fluorescence microscopy analysis of histone H3 staining confirmed this study ( Supplementary Fig. 3e,f ). Moreover, Trex1 −/− MEFs seemed to exhibit more histone H3 in the cytoplasm, as determined by this assay, compared with WT MEFs, even under untreated conditions ( Fig. 2e ; Supplementary Fig. 3e,f ). A similar effect was observed in MEFs lacking STING, again indicating that extranuclear nucleosome production does not require STING ( Fig. 2e ; Supplementary Fig. 3e,f ). Electron microscopy using gold-labelled antibody confirmed the presence of histones and dsDNA species in the cytoplasm of DMBA-treated MEF cells ( Fig. 2f ; Supplementary Fig. 3g,h ). The presence of histones/dsDNA was found to be increased in TKO MEFs treated with DMBA. However, even untreated TKO cells appeared to have slightly increased histone/dsDNA complexes in the cytoplasm compared with WT MEFs ( Fig. 2 ; Supplementary Fig. 3c–h ). Plausibly, Trex1 may function to help eliminate the presence of such leaked DNA into the cytoplasm. Collectively, our data indicate that DMBA may facilitate DNA leakage, a consequence that can lead to the activation of the STING pathway, an effect augmented by loss of Trex1. Figure 2: Cytoplasmic nucleosome production in DMBA-treated cells is independent of STING. ( a ) Fluorescence microscopy analysis of anti-dsDNA staining ( a , b ) and fluorescent in situ hybridization (FISH) with mouse centromere probe ( c , d ) in WT, TKO, STKO and SKO MEFs treated with DMBA at 20 μg ml − 1 or DMSO as control for 48 h. Representative images are shown at × 1,260; bar size, 10 μm ( a , c ), and ratio of cytoplasm to nucleus anti-dsDNA pixels from a and FISH pixels from c was quantitated using Leica LAS AF software ( b , d ). ( e ) Immunoblot analysis of histone H3 in cytoplasmic extraction from MEFs treated with DMBA same as in a or ultraviolet at 120 mJ cm − 2 followed by 24-h incubation (also see Supplementary Fig. 10 ). ( f ) Electron microscopy analysis of histone H3 and dsDNA gold staining in WT and TKO MEFs treated with DMBA same as in a . Arrows indicate gold particles in cytoplasm. Images were shown at original magnification, × 100,000; bar size, 100 nm. Data are representative of at least two independent experiments. Error bars indicate s.d. * P <0.05, *** P <0.001, Student’s t -test. Full size image STING − / − mice are resistant to DMBA skin tumorigenesis DMBA is used as a mutagen in tumorigenic studies and is known to induce inflammation-driven epithelial cancer when applied to the skin of mice, although the initiating pathway remains to be determined [2] , [9] . Given that we had observed that DMBA induces cytokine production in normal fibroblasts in a STING-dependent manner, we treated WT or STING-deficient mice (SKO) on a C57BL/6 background with 10 μg DMBA, orthotopically every week for 18 weeks. This study indicated that WT mice started to show tumour growth from the 7th week of DMBA treatment and about 90% of WT mice developed epithelial tumours (up to 6 tumours per mouse) at the end of the treatment period ( Fig. 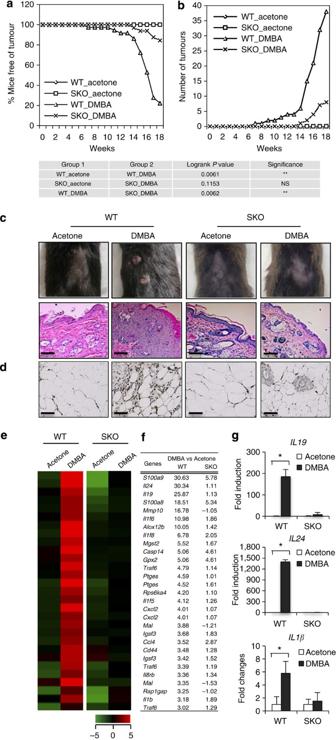Figure 3: DMBA-induced skin carcinogenesis is mediated through STING. (a) Percentage of skin-tumour-free mice and (b) number of skin tumours from DMBA-treated WT (n=18) and SKO mice (n=16). Acetone is used as control treatment. Results are shown in the Kaplan–Meier curve for the representative of two independent experiments.Pvalue of tumour incidence between group 1 and group 2 was calculated from the log-rank test. (c) Representative photographs of skin tumours and haematoxylin/eosin staining of the mice same as ina; all images were shown at original magnification, × 200; bar size, 200 μm. (d) CD68 immunohistochemistry staining of skin/tumours from mice same as ina; all images were shown at original magnification, × 400; bar size, 100 μm. (e) Gene array analysis of skin/tumour RNA isolated from the mice same as inaand (f) fold change values. Highest variable inflammation-related genes are shown. Rows represent individual genes; columns represent individual samples. Pseudo-colours indicate transcript levels below (green), equal to (black) or above (red) the mean. Scale represents the intensity of gene expression (log2 scale ranges between −5 and 5). (g) Quantitative PCR analysis ofIL19,IL24andIL1βfrom RNA same as ine. Data are the mean of three independent mice. Error bars indicate s.d. *P<0.05, Student’st-test. NS, not significant. 3a,b ; Supplementary Table 3 ). In contrast, fewer than 20% of SKO mice developed tumours within the same time period. Moreover, of those 20%, the number of tumours observed was <3 per animal and tumour growth was not observed until 14 weeks after DMBA treatment ( Fig. 3a,b ; Supplementary Table 3 ). Histological analysis of skin/tumour biopsies indicated that DMBA-treated WT mice developed squamous cell carcinoma (SCC) ( Fig. 3c ; Supplementary Fig. 4a ). CD68 and CD11c staining showed that DMBA-treated WT mice exhibited significant phagocytic infiltration and enhanced inflammation of the tumour/skin area ( Fig. 3d ; Supplementary Fig. 4b–d ). Indeed, the majority of DMBA-treated SKO mice showed no evidence of tumour presence or enhanced inflammation ( Fig. 3c,d ; Supplementary Fig. 4a–d ). To evaluate cytokine production in the skin of the treated WT or SKO mice, we performed DNA microarray analysis on tumours or skin derived from the treated animals. This study indicated extremely high levels of cytokine production in SCC derived from the DMBA-treated WT mice, including IL1β , IL24 , IL19 , IL6 and CCL5 , proinflammatory cytokines that have been shown to have profound effect in tumour development by numerous studies [21] , [22] , [23] ( Fig. 3e–g ; Supplementary Fig. 4e,f ). In contrast, the levels of these cytokines were significantly ablated in the skin of similarly treated SKO mice or mock-treated control mice ( Fig. 3e–g ; Supplementary Fig. 4e,f ). Our data demonstrate that STING-dependent cytokine production is responsible for DMBA-dependent inflammatory carcinogenic disease. We similarly treated Trex1-deficient mice (TKO) with DMBA. All DMBA-treated TKO mice developed skin tumours as early as 9 weeks. Histological analysis of the skin derived from treated TKO mice showed markedly thickened epidermis with SCC extending into the dermis ( Supplementary Fig. 5 ). Langerhans cells (LCs) have been reported to play a key role in manifesting DMBA-facilitated inflammatory tumours [24] , [25] . We observed that, upon DMBA treatment, WT skin/tumour showed a notable increase in LCs (using CD207 antibody) compared with SKO skin ( Supplementary Fig. 6a,b ). We also evaluated DMBA metabolic profile in WT versus SKO MEFs by high-pressure liquid chromatography (HPLC). Our data suggested that both MEFs are capable of metabolizing DMBA, which is consistent with the comparable level of DNA damage observed in DMBA-treated WT and SKO MEFs ( Supplementary Fig. 6c ). Thus, DNA-damage-induced inflammatory carcinogenesis can be facilitated through the STING pathway. Figure 3: DMBA-induced skin carcinogenesis is mediated through STING. ( a ) Percentage of skin-tumour-free mice and ( b ) number of skin tumours from DMBA-treated WT ( n =18) and SKO mice ( n =16). Acetone is used as control treatment. Results are shown in the Kaplan–Meier curve for the representative of two independent experiments. P value of tumour incidence between group 1 and group 2 was calculated from the log-rank test. ( c ) Representative photographs of skin tumours and haematoxylin/eosin staining of the mice same as in a ; all images were shown at original magnification, × 200; bar size, 200 μm. ( d ) CD68 immunohistochemistry staining of skin/tumours from mice same as in a ; all images were shown at original magnification, × 400; bar size, 100 μm. ( e ) Gene array analysis of skin/tumour RNA isolated from the mice same as in a and ( f ) fold change values. Highest variable inflammation-related genes are shown. Rows represent individual genes; columns represent individual samples. Pseudo-colours indicate transcript levels below (green), equal to (black) or above (red) the mean. Scale represents the intensity of gene expression (log2 scale ranges between −5 and 5). ( g ) Quantitative PCR analysis of IL19 , IL24 and IL1β from RNA same as in e . Data are the mean of three independent mice. Error bars indicate s.d. * P <0.05, Student’s t -test. NS, not significant. Full size image STING in bone marrow contributes to DMBA skin tumorigenesis To evaluate the role of hematopoietic cells (plausibly antigen-presenting cells) in DMBA-induced carcinogenesis, we irradiated 8-week-old WT or SKO mice and adoptively transferred them with bone marrow from WT or SKO mice. The transplanted mice were then treated with or without DMBA 28 days later for up to 20 weeks. This study showed that DMBA-treated WT mice previously transplanted with WT bone marrow exhibited a similar frequency of developing epithelial carcinoma compared with WT mice treated with DMBA alone (up to 9 tumours per mouse) ( Fig. 4a–d ). In contrast, WT mice transplanted with bone marrow obtained from SKO mice developed fewer tumours (<2 tumours per mouse), with >60% of the animals remaining tumour free ( Fig. 4c,d ). It is plausible that the persistence of tumour development in some of the SKO bone-marrow-transferred WT mice is due to DMBA-induced cytokine production in radioresistant cells (for example, LCs, keratinocytes and so on) that are still positive for STING. More significantly, irradiated SKO mice treated with DMBA after transplantation with bone marrow from WT mice developed tumours to a similar frequency compared with irradiated, DMBA-treated WT mice receiving WT bone marrow ( Fig. 4c,d ). Histological examination indicated that both WT and SKO mice transplanted with WT bone marrow developed severe SCC, whereas the majority of WT and all SKO mice transplanted with SKO bone marrow showed no tumour or inflammation ( Fig. 4e ). Thus, we conclude that while carcinogen-treated fibroblasts or epithelial cells are able to recognize DNA damage and produce cytokines in a STING-dependent manner, it is likely that this event promotes the infiltration of phagocytes. These latter cells encounter the DNA-damaged cells and engulf them [3] , [5] . This event triggers further STING-dependent cytokine production, which predominantly drives inflammation-dependent tumorigenesis. Indeed, our studies indicated that macrophages more readily engulfed DMBA-treated cells compared with untreated cells, an effect that could stimulate cytokine production ( Supplementary Fig. 7 ). A key objective for the future would include identifying which cells (that is, tissue resident keratinocytes or inflammatory residual dendritic cells, LCs or macrophages) are predominantly involved in STING-dependent cytokine production and skin tumorigenesis. This will require confirming which cells are involved in DMBA metabolism and discerning between tumour induction by such agents and the promotion of cancer by the inflammatory response. 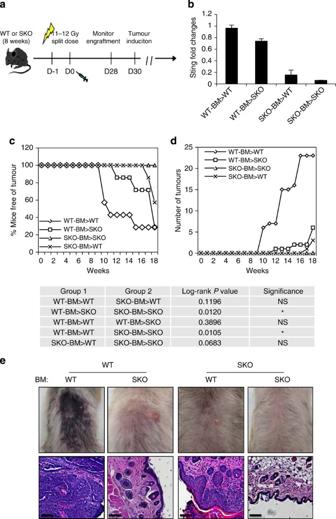Figure 4: STING in hematopoietic cells contributes to DMBA-induced carcinogenesis. (a) Schematic representation of bone marrow transplantation (BMT). (b) STING expression level in peripheral blood mononucleated cell 4 weeks post BMT. Transplant groups are labelled as: donor bone marrow>recipient. (c) Percentage of skin-tumour-free mice and (d) number of skin tumours from DMBA-treated mice previously transplanted with bone marrow as indicated.N=7 per group. Results are shown in the Kaplan–Meier curve.Pvalue of tumour incidence between group 1 and group 2 was calculated from the log-rank test. (e) Representative photographs of skin tumours and haematoxylin/eosin staining of the mice same as inc. Images are shown at original magnification, × 200; bar size, 200 μm. NS, not significant. Figure 4: STING in hematopoietic cells contributes to DMBA-induced carcinogenesis. ( a ) Schematic representation of bone marrow transplantation (BMT). ( b ) STING expression level in peripheral blood mononucleated cell 4 weeks post BMT. Transplant groups are labelled as: donor bone marrow>recipient. ( c ) Percentage of skin-tumour-free mice and ( d ) number of skin tumours from DMBA-treated mice previously transplanted with bone marrow as indicated. N =7 per group. Results are shown in the Kaplan–Meier curve. P value of tumour incidence between group 1 and group 2 was calculated from the log-rank test. ( e ) Representative photographs of skin tumours and haematoxylin/eosin staining of the mice same as in c . Images are shown at original magnification, × 200; bar size, 200 μm. NS, not significant. Full size image Our data thus indicate that chronic exposure to carcinogens that induce DNA adduct formation and breakage can cause nucleosome leakage and trigger cytosolic DNA signalling that is dependent on STING. This effect is greatly augmented in the absence of Trex1 (DNaseIII), indicating a possible role for this predominantly ER-associated exonuclease in eliminating self-DNA that has leaked into the cytoplasm, consequences that lead to the enhanced stimulation of STING ( Supplementary Fig. 8 ). Loss of TNFα or MyD88 has also been shown to render mice resistant to DMBA treatment [11] , [12] . However, we have found that STING-dependent primary innate immune gene activation remains intact in MyD88 lacking MEFs ( Supplementary Fig. 9 ). Thus, STING likely triggers the expression of select cytokines that in turn bind receptors requiring MyD88 signalling for the production of proinflammatory cytokines such as TNFα [2] . It is also plausible that drugs such as cisplatin and etoposide, given transiently, may exert some of their anti-tumour activity by triggering STING-dependent innate immune activity. These events could facilitate tumour clearance by stimulating anti-tumour-adaptive immune responses. It is further tempting to speculate that stimuli such as PAHs, that are predominant in numerous environmental toxins such as smoke and certain foods, could play a role, at least in part, for the inflammatory effects observed in patients with defects in genes such as Trex1, which can cause lethal AGS or less-severe types of SLE. Our data, which is the first report for a role of the STING pathway in cancer, suggest that controlling STING-dependent cytokine production could have beneficial effects on the outcome of certain malignant diseases. Thus, therapeutics that control STING may provide a new generation of anti-cancer treatments. Materials All cell culture media or reagents were from Invitrogen unless specified. All chemicals were from Sigma unless specified. Mice SKO mice were generated in our laboratory (Ishikawa et al . [13] ). Trex1 hetero mice (Trex1 +/ − ) were kindly provided by Dr Lindahl and Barnes (London Research Institute). SKO mice were crossed with Trex1 +/ − mice to generate STING and Trex1 double-knockout mice (STKO). Mice care and study were conducted under approval from the Institutional Animal Care and Use Committee of the University of Miami. Mouse genotypes from tail biopsies were determined by using real-time PCR with specific probes designed for each gene by commercial vendor (Transnetyx). Mouse treatment Dorsal skin 1–2 cm 2 of 8-week-old female mice was shaved. For treatment with DMBA, 10 μg of DMBA in 100 μl of acetone was applied to shaved skin once per week for 18–20 weeks. Acetone (100 μl) was applied to control groups. Tumour development was assessed weekly. A mouse was killed if tumours reached 1 cm in any diameter or became obviously invasive or ulcerated. Skin/tumour biopsies were stored or treated for specific applications. Immunohistochemistry and histological analysis Skin/tumour biopsies were fixed with 10% formalin for 72 h and tranferred to 70% ethanol for long-time storage. Haematoxylin/eosin staining and immunohistochemistry staining of CD68 (AbD Serotec) at 1:200 dilution were done by IHC world. CD207 (Thermo Scientific) at 1:200 dilution and CD11c at 1:400 dilution (Bioss USA) staining and histological examination were performed by Dr Phillip Ruiz. Bone marrow transplantation Bone marrow cells were primarily harvested from the long bones of donor mice by flushing with a 26-gauge needle. Single-cell suspensions were T-cell depleted using anti-Thy1.2 (HO-13.4 supernatant) antibody at 1:5 vol/vol for 30 min on ice, followed by addition of 12% Low-Tox M rabbit complement (Cedarlane Labs), incubated at 37 °C for 1 h. Depletion efficiency was routinely >95%. Recipient mice were lethally irradiated with a 137 Cs source at 6.5 Gy each 1 day before (day −1) and on the day of transplantation (day 0), and later injected intravenously with 1 × 10 6 T-cell-depleted bone marrow cells. Hematopoietic cell population was examined by flow cytometry 4 weeks later to ensure engraftment. Transplanted mice were then treated with DMBA as described. Primary cells and drug treatments Mouse embryonic fibroblasts (MEFs) were obtained from e13.5 embryos by a standard procedure. Normal human epidermal keratinocytes and culture media were purchased from Lonza. Unless specified, cells were treated with DMBA at 20 μg ml − 1 , cisplatin at 10 μM or etoposide at 250 μM for 48 h. Dimethyl sulfoxide (DMSO) was used for control treatment. Ultraviolet treatment on MEFs was performed in a UVC500 UV crosslinker at 120 mJ cm −2 followed by 24-h incubation. Gene array analysis Total RNA was isolated from cells or tissues using the RNeasy Mini kit (Qiagen). RNA quality was analysed using the Bionalyzer RNA 6000 Nano (Agilent Technologies). Gene array analysis was examined using the Illumina Sentrix BeadChip Array (Mouse WG6 version 2) at the Oncogenomics Core Facility, University of Miami. Gene expression profiles were processed and statistical analysis was performed at the Bioinformatics Core Facility, University of Miami. Briefly, raw intensity values from the Illumina array are uploaded on GeneSpring software from Agilent. Values are Quantile normalized and log2-transformed to the median of all samples. Significantly differential expressed genes from a two-class comparison are computed using the Student’s t -test and selected using a threshold of P -value ≤0.05. Hierarchical clustering and visualization of selected differentially expressed genes is performed on GeneSpring using the Pearson correlation distance method, and linkage was computed using the Ward method. Fold change analysis was performed between two groups and differentially expressed genes were selected based on threshold of fold changes. Cytoplasmic nucleosome detection The cytoplasmic fraction was extracted from DMBA-treated MEFs using NE-PER nuclear and cytoplasmic extraction reagents (Thermo scientific). Equal amounts of proteins were analysed by immunoblot. ELISA IFNβ levels were determined from cell culture supernatant using the VeriKine Mouse IFN-Beta ELISA Kit (PBL IFN Source) following the manufacturer’s instruction. Quantitative real-time PCR Total RNA was reverse-transcribed using the QuantiTect Reverse Transcription Kit (Qiagen). Real-time PCR was performed with the TaqMan gene Expression Assay (Applied Biosystems). mSTING-S (5′- CATTGGGTACTTGCGGTT -3′), mSTING-AS (5′- CTGAGCATGTTGTTATGTAGC -3′), mMyd88-S (5′- CACCAAGTCCTGGTTCTGG -3′) mMyd88-AS (5′- TAGACAGGACGGCATCAGAG -3′) was used for Sybr green analysis. Taqman gene expression assay: mouse CXCL10, Mm00445235; human CXCL10, Hs00171042; mouse IFNB, Mm00439552; Human IFNB, Hs00277188; mouse IL6, Mm00446190; mouse IL1B, Mm01336189; mouse cGAS, Mm01147497; mouse IL19, Mm01288324; mouse IL24, Mm00474102; mouse IRF1, Mm01288580, mouse TNFalpha, Mm00443258; mouse IRF7, Mm00516788; mouse CCL5, m01302427. Immunofluorescence staining Cells were fixed with 4% paraformaldehyde in Dulbecco's modified Eagle's medium for 15 min at 37 °C and were permeabilized with 0.2% Triton X-100. Fixed and permeabilized cells were blocked with 10% bovine serum albumin in phosphate-buffered saline, incubated with primary antibodies in 2% bovine serum albumin in phosphate-buffered saline and then incubated with fluorophore-conjugated secondary antibodies (with 4′,6-diamidino-2-phenylindole (DAPI) counterstaining). After staining, cells were mounted in anti-fade mounting solution (Invitrogen) and examined under a Leica SP5 spectral confocal inverted microscope. Antibodies used including HA (Sigma) at 1:200 dilution, calreticulin (Abcam) at 1:200 dilution, IRF3 (Santa cruz) at 1:200 dilution, p65 (Cell signaling) at 1:200 dilution, dsDNA (Abcam) at 1:500 dilution and Histone H3 (Abcam) at 1:500 dilution. PicoGreen staining PicoGreen staining was performed using Quant-iT PicoGreen dsDNA reagent and kits from Invitrogen. For confocal microscopy, cells were incubated in the presence of PicoGreen at 37 °C for 1 h, washed and fixed for confocal microscopy with DAPI counterstaining. Electron microscopy After treatment, MEF cells were fixed in 4% paraformaldehyde. Histone H3 (Abcam, at 1:50 dilution) and dsDNA (Abcam, at 1:50 dilution) gold staining and electron microscopy analysis were performed by the electron microscopy core facility at Miami Project to Cure Paralysis, University of Miami Miller School of Medicine. Fluorescence in situ hybridization Cells were seeded on coverslips and treated appropriately. Fluorescence in situ hybridization was performed using the Cytology FISH accessory kit from DAKO following the manufacturer’s instruction. Fluorescein isothiocyanate-labelled all-mouse centromere probe was purchased from Kreatech Diagnostics. Bone marrow macrophage isolation and in vitro phagocytosis Bone marrow macrophages were isolated from hind-limb femurs of 8-week-old WT and SKO mice. Briefly, the marrow cells were flushed from the bones with alpha minimum essential medium supplemented with 10% heat-inactivated foetal calf serum with a 26-gauge needle and incubated at 37 °C for 4 h. Approximately 2 × 10 7 cells were seeded in a 10-cm dish with complete alpha minimum essential medium including 10 ng ml − 1 of mouse recombinant colony-stimulating factor (M-CSF, 416-ML) (R&D Systems). After 1 week, bone marrow-derived macrophages were obtained. In vitro phagocytosis was performed as described by Ahn et al . [5] . Specifically, thymocytes were isolated from 8-week-old mice, treated with 20 μg ml − 1 of DMBA for 48 h and transfected with fluorescein isothiocyanate-labelled dsDNA and then added to macrophages for 1 h. Following vigorous washing to remove unengulfed thymocytes, macrophages were fixed with 4% paraformaldehyde solution overnight at 4 °C, counterstained with DAPI and subjected to fluorescence microscopy analysis. For gene expression, macrophages were incubated with thymocytes for 6 h and subjected to quantitative PCR analysis. Immunoblot analysis Equal amounts of proteins were resolved on SDS-polyacrylamide gels and then transferred to polyvinylidene fluoride membranes (Millipore). After blocking with 5% Blocking Reagent, membranes were incubated with various primary antibodies (and appropriate secondary antibodies). The image was resolved using an enhanced chemiluminescence system ECL (Thermo Scientific) and detected by autoradiography (Kodak). Antibodies: rabbit polyclonal antibody against STING was developed in our laboratory as described previously (Ishikawa et al . [6] ); other antibodies were obtained from following sources: HA (Sigma Aldrich, at 1:10,000 dilution), β-actin (Sigma Aldrich, at 1:10,000 dilution), p-IRF3 (Cell Signaling, at 1:1,000 dilution), p-p65 (Cell Signaling at 1:1,000 dilution), p65 (Cell Signaling at 1:1,000 dilution), IRF3 (Santa Cruz Biotechnology, at 1:1,000 dilution), Histone H3 (Abcam at 1:1,000 dilution) and MyD88 (Abcam, at 1:500 dilution). HPLC analysis of DMBA metabolism Medium from treated MEFs as well as controls were collected and extracted with three equal volume of ethyl acetate. The organic extracts were evaporated to dryness with a Savant SpeedVac Evaporator/Concentrator. The pH of the remaining aqueous fraction was lowered to 2.5 with 6 M hydrochloric acid, and the contents were extracted again with ethyl acetate to isolate the acidic metabolites. The residues were dissolved in 30% methanol for analysis by reversed-phase HPLC. DMBA and its metabolites were separated by HPLC using the Agilent Infinity 1260 LC system with a ZORBAX SB-C18 3.5-Micron 4.6 × 150 mm column (Agilent) at a flow rate of 1 ml min −1 . The compounds were eluted with a linear gradient of 40–95% methanol–water over 50 min. Statistical analysis All statistical analyses were performed by the Student’s t -test unless specified. The data were considered to be significantly different when P <0.05. How to cite this article: Ahn, J. et al . Inflammation-driven carcinogenesis is mediated through STING. Nat. Commun. 5:5166 doi: 10.1038/ncomms6166 (2014). Accession codes: Gene array data has been deposited to GEO (Accession number GSE57605 ).